IL-27 and IL-12 oppose pro-inflammatory IL-23 in CD4+T cells by inducing Blimp1 Central nervous system (CNS) autoimmunity is regulated by the balance of pro-inflammatory cytokines and IL-10. Here we identify the transcriptional regulator Blimp1 as crucial to induce IL-10 in inflammatory T helper cells. Pre-committed Th17 cells respond to IL-27 and IL-12 by upregulating Blimp1 and adopt a Tr-1-like phenotype characterized by IL-10 and IFN-γ production. Accordingly, Blimp1-deficient effector T cells fail to produce IL-10, and deficiency in Tr-1 cell function leads to uncontrolled Th17 cell-driven CNS pathology without the need to stabilize the Th17 phenotype with IL-23. IL-23 counteracts IL-27 and IL-12-mediated effects on Tr-1-development reinforcing the pro-inflammatory phenotype of Th17 cells. Thus, the balance of IL-23 vs IL-12/IL-27 signals into CD4 + effector T cells determines whether tissue inflammation is perpetuated or resolves. Th1, Th2, Th17 and T follicular helper cells have been defined as effector T helper cell lineages based on distinct signature cytokines as well as master transcription factors that control their development from naive CD4 + precursor T cells [1] , [2] , [3] . While the cytokine phenotypes of IFN-γ-producing Th1 cells and IL-4-producing Th2 cells are relatively stable [4] , Th17 cells appear to be more plastic [5] , [6] , [7] . This may be due to the activity of TGF-β, which inhibits premature commitment of naive CD4 + T cells and allows for the T-cell extrinsic cytokines IL-6 and IL-27 to promote the induction of IL-17 (Th17 cells) and IL-10 (Tr-1 cells), respectively [8] , [9] . Although it has been suggested that Tr-1 cells represent a distinct T helper cell lineage [10] , [11] , their phenotype and transcription factor requirements, in particular in vivo , are not well known. IL-10-producing CD4 + T cells have increasingly been reported in the target tissue of viral or parasitic infections [12] , [13] , and CD4 + T cells of this particular phenotype were also detected in humans [14] . Most of these effector T cells were IL-10/IFN-γ double producers, and it is a matter of debate and definition whether these T cells are ‘Tr-1’ cells. Indeed, rather than initial commitment of naive CD4 + T cells to a distinct Tr-1 lineage, acquisition of the ability to produce IL-10 may also result from T-cell plasticity or re-programming [15] . Thus, distinct molecular mechanisms may exist that instruct IL-10 production in effector T cells. In addition to c-Maf and Ahr [16] , the transcriptional regulator B lymphocyte-induced maturation protein-1 (Blimp1) has recently been implicated in IL-10 production from Tr-1 cells [17] . Blimp1 is a zinc-finger protein, which is transcribed from the Prdm1 gene [18] . It is required for the differentiation of B cells into plasma cells [19] , [20] and has critical roles in the homeostasis and function of various T-cell populations [21] , [22] . Importantly, the production of IL-10 by effector CD8 + and Foxp3 + regulatory T cells (Tregs) requires the expression of Blimp1 (refs 23 , 24 ). Autoimmune inflammation in the central nervous system (CNS) is largely driven by IL-23-‘stabilized’ Th17 cells [25] , [26] and IL-23R-deficient mice are resistant to experimental autoimmune encephalomyelitis (EAE) [27] , [28] . Here, we observed that resistance to EAE of IL-23R-deficient mice is correlated with exaggerated generation of IL-10/IFN-γ double producing T cells. Thus, we hypothesized that a major function of IL-23 might be to prevent Th17 cells from adopting an IL-10/IFN-γ-producing phenotype. When comparing the gene expression profile of Th17 cells and Tr-1 cells, we found that Blimp1 was highly expressed in Tr-1 cells but not in Th17 cells. Notably, our analysis revealed that committed Th17 cells were not only able to respond to IL-23 (p19/p40) but also to IL-27 (p28/EBI3) and IL-12 (p35/p40). While IL-23 promoted the maintenance of IL-17 production and did not induce Blimp1 in committed Th17 cells, IL-27 was a strong inducer of Blimp1, which prompted Th17 cells to switch to the production of large amounts of IL-10. IL-12 could in part substitute for IL-27 in this function. We therefore propose a model, in which the balance of IL-27 and IL-12 vs IL-23 signalling in CD4 + T cells is critical for the development of suppressive IL-10-producing Tr-1-like cells or pathogenic Th17 cells, respectively. IL-23 is dispensable for EAE in Ifng −/− × Il-10 −/− mice When Th17 cells were first proposed as a lineage of their own in 2005, IFN-γ was shown to inhibit their development [29] , [30] . Moreover, Th17 cells that are differentiated in the presence of TGF-β plus IL-6 have been regarded as non-pathogenic in part because they also produced IL-10 (ref. 31 ). In contrast, IL-23 has been considered as the one non-redundant factor required for the induction of immunopathology in T helper cell-mediated models of autoimmunity and chronic inflammation because it induced GM-CSF in T helper cells in a Ror-γt-dependent manner [32] , [33] . Here, we wanted to revisit whether IL-23 was indeed indispensable for conferring pathogenic properties to effector T helper cells and induce Th17-mediated autoimmunity. We decided to apply a genetic approach by using the EAE resistant Il23r −/− strain and in addition, introduced deficiency of Ifng or Il-10 , or disrupted both genes by crossing Il-10 −/− and Ifng −/− mice into the Il23r −/− background. While Il23r +/− mice developed a disease phenotype similar to wild-type animals and Il23r −/− mice were resistant to EAE as expected, disruption of either Il-10 or Ifng on the Il23r −/− background failed to break resistance to disease. In contrast, double deficiency of IL-10 and IFN-γ rendered Il23r −/− mice hypersusceptible to EAE and unable to control CNS inflammation ( Fig. 1a,b ). Since pathogenic effector T helper cells are not believed to be inducible in the absence of IL-23 signalling, we investigated the cytokine phenotype of conventional CD4 + T helper cells isolated from the inflamed CNS of triple KO mice ( Fig. 1c ). Triple KO CD4 + effector T cells produced IL-17 and large amounts of GM-CSF. Comparing all IL-23R-deficient experimental groups, any combination of IL-17 and GM-CSF was less of a predictor of immunopathology than the presence or absence of IL-10 and IFN-γ-producing CD4 + T cells in the CNS. Thus, the abundance of IL-10/IFN-γ producers in the conventional T-cell compartment correlated with the extent of resistance to the tissue inflammation in Il23r −/− mice. This observation was surprising and prompted us to re-investigate the paradigm of pathogenic vs non-pathogenic Th17 cells on a molecular level [34] . We focused on Th17 cells because Th1 cells did not express the IL-23R anyway ( Supplementary Fig. 1 ) and were thus unlikely to be affected by the disruption of the Il23r gene. 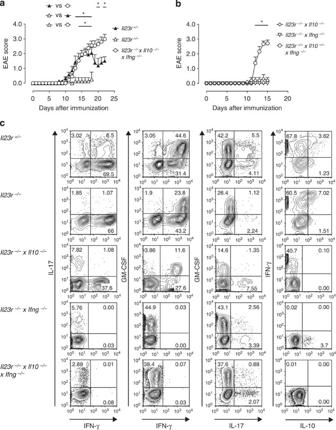Figure 1: IL-23 is dispensable for CNS immunopathology in the absence of IFN-γ and IL-10. (a,b)Il23r+/−(control) mice,Il23r−/−mice,Il23r−/−× Il-10−/−mice,Il23r−/−× Ifng−/−mice, or triple deficientIl23r−/−× Il-10−/−× Ifng−/−mice were immunized according to the standard EAE induction protocol. Mean clinical scores ±s.e.m. are shown. Representative of three experiments withn≥3, *P<0.05, two-way analysis of variance. (c) At the peak of disease (d18 to d20), mononuclear cells were isolated from the CNS and intracellular cytokine staining was performed. Fractions of IL-17 vs IFN-γ, GM-CSF vs IFN-γ, GM-CSF vs IL-17, and IL-10 vs IFN-γ expressing cells within the conventional CD4+T cell gate are shown (representative cytograms out of three). Figure 1: IL-23 is dispensable for CNS immunopathology in the absence of IFN-γ and IL-10. ( a , b ) Il23r +/− (control) mice, Il23r −/− mice, Il23r −/− × Il-10 −/− mice, Il23r −/− × Ifng −/− mice, or triple deficient Il23r −/− × Il-10 −/− × Ifng −/− mice were immunized according to the standard EAE induction protocol. Mean clinical scores ±s.e.m. are shown. Representative of three experiments with n ≥3, * P <0.05, two-way analysis of variance. ( c ) At the peak of disease (d18 to d20), mononuclear cells were isolated from the CNS and intracellular cytokine staining was performed. Fractions of IL-17 vs IFN-γ, GM-CSF vs IFN-γ, GM-CSF vs IL-17, and IL-10 vs IFN-γ expressing cells within the conventional CD4 + T cell gate are shown (representative cytograms out of three). Full size image Blimp1 expression is a hallmark of IL-10 + IFN-γ + T cells Since we found that Il-10 −/− × Ifng −/− mice developed severe EAE in the absence of IL-23 signalling ( Fig. 1 ), we raised the hypothesis that one essential function of IL-23 would be to suppress IL-10 and IFN-γ in T cells. Therefore, we designed an experimental approach to identify transcriptional regulators in T cells that were associated with an IL-10 and IFN-γ double producing phenotype. IL-27 together with low amounts of TGF-β was reported to induce IL-10 and IFN-γ producing CD4 + T cells in vitro [9] , [35] . Thus, we asked the question which transcription factors were differentially expressed in these so-called Tr-1 cells as compared with Th17 cells that were differentiated with IL-6 and TGF-β and had not yet sensed IL-23. Using this strategy, we expected to identify factors that were responsible for inducing the IL-10/IFN-γ transcriptional module which—if absent in T cells—allowed for the generation of pathogenic Th17 cells without sensing IL-23. When we interrogated a microarray expression analysis of in vitro -differentiated Tr-1 vs Th17 cells, the most prominently overexpressed transcription factors in Tr-1 cells vs Th17 cells included Irf1 , Irf8, Prdm1 (termed Blimp1 hereafter) and Tbx21 ( Fig. 2a ; Supplementary Tables 1,2 ). Since Blimp1 is required for the expression of IL-10 in CD8 + T cells and Tregs [23] , [24] , we sought to examine the functional relevance of Blimp1 in Tr-1 cells. First, we confirmed by quantitative PCR analysis and Blimp1 reporter T cells ( Blimp1 gfp/+ ) that Blimp1 messenger RNA was significantly higher expressed in Tr-1 than in Th17 cells ( Fig. 2b,c ). Importantly, western blot analysis showed that similar to Th1 cells, Tr-1 cells expressed high amounts of Blimp1 protein whereas Th17 cells lacked Blimp1 ( Fig. 2d ). Notably, Blimp1 expression was highest in the IL-10/IFN-γ double producing Tr-1 cells ( Fig. 2e ). 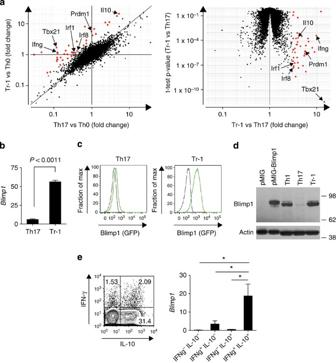Figure 2:The transcriptional regulator Blimp1 is required for IL-27 mediated IL-10 induction in CD4+T cells. (a) Naive CD4+T cells were polyclonally stimulated for 3 days with plate-bound antibody to CD3 and soluble antibody to CD28 in the absence of exogenous cytokines (Th0), or differentiated into Tr-1 cells (100 ng ml−1IL-27 plus 0.5 ng ml−1TGF-β) or Th17 cells (50 ng ml−1IL-6 plus 0.5 ng ml−1TGF-β) for microarray analysis (Affymetrix). Mean expression values of five independent experiments are depicted as fold change Tr-1/Th0 (Yaxis) vs fold change Th17/Th0 (Xaxis), left, and fold change Tr-1/Th17 vst-testP-value (volcano plot), right. Genes with at least threefold higher expression in Tr-1 cells as compared with Th17 cells are highlighted in red. (b) Relative messenger RNA abundance ofBlimp1in Th17 cells vs Tr-1 cells as measured by quantitative RT–PCR. Mean±s.d., four experiments withn=3, two-tailedt-test. (c) Expression ofBlimp1in Tr-1 cells and Th17 cells differentiated from naiveBlimp1gfp/+(green line) or wild-type (black line) CD4+T cells as measured by flow cytometry. Representative cytograms out of three independent experiments. (d) Blimp1 protein expression in Th1 cells, Th17 cells and Tr-1 cells as measured by western blot (positive control: overexpressed Blimp1 in retrovirally transduced naive T cells). Representative blot out of three experiments. (e) Naïve CD4+T cells from wild-type mice were differentiated into Tr-1 cells. On day 3, cells were FACS sorted according to their expression of IL-10 and/or IFN-γ and assayed forBlimp1expression by qPCR. Representative of three similar experiments, mean±s.d.,n=3, *P<0.05, one-way analysis of variance followed by Tukey post test. Figure 2: The transcriptional regulator Blimp1 is required for IL-27 mediated IL-10 induction in CD4 + T cells. ( a ) Naive CD4 + T cells were polyclonally stimulated for 3 days with plate-bound antibody to CD3 and soluble antibody to CD28 in the absence of exogenous cytokines (Th0), or differentiated into Tr-1 cells (100 ng ml −1 IL-27 plus 0.5 ng ml −1 TGF-β) or Th17 cells (50 ng ml −1 IL-6 plus 0.5 ng ml −1 TGF-β) for microarray analysis (Affymetrix). Mean expression values of five independent experiments are depicted as fold change Tr-1/Th0 ( Y axis) vs fold change Th17/Th0 ( X axis), left, and fold change Tr-1/Th17 vs t -test P -value (volcano plot), right. Genes with at least threefold higher expression in Tr-1 cells as compared with Th17 cells are highlighted in red. ( b ) Relative messenger RNA abundance of Blimp1 in Th17 cells vs Tr-1 cells as measured by quantitative RT–PCR. Mean±s.d., four experiments with n =3, two-tailed t -test. ( c ) Expression of Blimp1 in Tr-1 cells and Th17 cells differentiated from naive Blimp1 gfp/+ (green line) or wild-type (black line) CD4 + T cells as measured by flow cytometry. Representative cytograms out of three independent experiments. ( d ) Blimp1 protein expression in Th1 cells, Th17 cells and Tr-1 cells as measured by western blot (positive control: overexpressed Blimp1 in retrovirally transduced naive T cells). Representative blot out of three experiments. ( e ) Naïve CD4 + T cells from wild-type mice were differentiated into Tr-1 cells. On day 3, cells were FACS sorted according to their expression of IL-10 and/or IFN-γ and assayed for Blimp1 expression by qPCR. Representative of three similar experiments, mean±s.d., n =3, * P <0.05, one-way analysis of variance followed by Tukey post test. Full size image In the presence of high amounts of TGF-β, we found that IL-27-driven IL-10 expression was largely independent of Blimp1 ( Fig. 3a,b ) and might rely on other transcription factors like c-Maf and Ahr ( Fig. 3a ) that were previously implicated in the induction of Il-10 (refs 16 , 36 ). However, in the absence of TGF-β, IL-27 failed to promote IL-10 production in Blimp1-deficient CD4 + T cells ( Fig. 3b ). Thus, our data indicated that IL-27 was sufficient to induce Blimp1 and sustain high IL-10 expression. As Th1 cells expressed Blimp1 ( Fig. 2d ), we wished to test whether IL-12 could substitute for IL-27 in the induction of Blimp1-mediated IL-10 expression. Indeed, Blimp1 expression was absolutely required for IL-12 to induce IL-10 in activated CD4 + T cells ( Fig. 3b ). In contrast to IL-27-induced Tr-1 cells and IL-12-induced Th1 cells, IL-10 production was Blimp1 independent in Th2 cells and Th17 cells that were differentiated in the presence of TGF-β plus IL-6 ( Fig. 3c ). 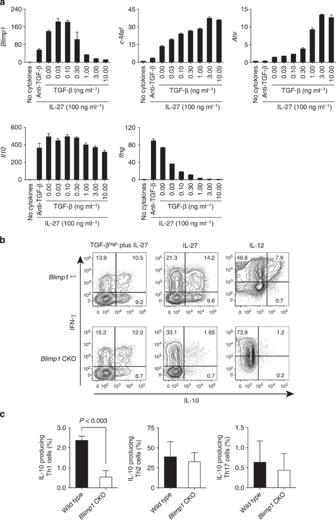Figure 3:Blimp1 is necessary for IL-27 to induce IL-10 in naive CD4+T cells in the absence of TGF-β. (a) Naive CD4+T cells were differentiated by activation with plate-bound anti-CD3 and soluble anti-CD28 with IL-27 alone (in the presence of a blocking antibody to TGF-β) or with IL-27 in the presence of increasing concentrations of TGF-β. Quantification of the indicated messenger RNAs was performed by quantitative RT–PCR on day 3. Mean±s.d.,n=3, representative of three experiments. (b) Naive CD4+T cells from control mice (Blimp1+/+) or T cell conditional Blimp1-deficient mice (Blimp1CKO) were differentiated in the presence of the indicated cytokines followed by intracellular cytokine staining on day 4 of culture. Representative of three independent experiments. (c) CD4+T cells from control orBlimp1CKO mice were differentiatedin vitrointo Th1 cells (IL-12 plus anti-IL-4), Th2 cells (IL-4 plus anti-IL-12) and Th17 cells (TGF-β plus IL-6) and assessed for intracellular cytokines on day 4. Frequencies of IL-10+producing T cells are depicted. Mean±s.d.,n=3, two-tailedt-test; representative of three experiments. Figure 3: Blimp1 is necessary for IL-27 to induce IL-10 in naive CD4 + T cells in the absence of TGF-β. ( a ) Naive CD4 + T cells were differentiated by activation with plate-bound anti-CD3 and soluble anti-CD28 with IL-27 alone (in the presence of a blocking antibody to TGF-β) or with IL-27 in the presence of increasing concentrations of TGF-β. Quantification of the indicated messenger RNAs was performed by quantitative RT–PCR on day 3. Mean±s.d., n =3, representative of three experiments. ( b ) Naive CD4 + T cells from control mice ( Blimp1 +/+ ) or T cell conditional Blimp1-deficient mice ( Blimp1 CKO) were differentiated in the presence of the indicated cytokines followed by intracellular cytokine staining on day 4 of culture. Representative of three independent experiments. ( c ) CD4 + T cells from control or Blimp1 CKO mice were differentiated in vitro into Th1 cells (IL-12 plus anti-IL-4), Th2 cells (IL-4 plus anti-IL-12) and Th17 cells (TGF-β plus IL-6) and assessed for intracellular cytokines on day 4. Frequencies of IL-10 + producing T cells are depicted. Mean±s.d., n =3, two-tailed t -test; representative of three experiments. Full size image Collectively our data indicated that Blimp1 was intrinsically required for IL-10 production in CD4 + T cells activated in the presence of IL-27 or IL-12. Furthermore, this dependence on Blimp1 was circumvented by high amounts of TGF-β. IL-27 and IL-12 induce IL-10 in Th17 cells via Blimp1 Our in vitro differentiation cultures were always started with sorted naive (CD44 − CD62L high ) T cells. We wondered whether IL-27 or IL-12 were also sufficient to re-programme pre-committed Th17 cells. Thus, we differentiated Th17 cells from naive wild-type T cells and sorted actual IL-17 producers by MACS bead secretion assay. The expression of the receptors for IL-27 and IL-12 suggested that IL-17 + Th17 cells were potentially responsive to both IL-27 and IL-12 ( Fig. 4a ). The IL-12 and IL-27 receptor expression profiles in sorted IL-17 + Th17 cells closely resembled the cytokine receptor expression profile in ex vivo -sorted bona fide (IL-23R + ) Th17 cells from EAE mice ( Fig. 4b ). When purified IL-17 + Th17 cells were re-stimulated in the presence of IL-12 family cytokines, both IL-27 and IL-12 induced the expression of Blimp1 ( Fig. 4c,d ) and enhanced the secretion of IL-10 and IFN-γ ( Fig. 4e,f ; Supplementary Fig. 2 ). In contrast, IL-23 failed to induce Blimp1 but stabilized the expression of IL-17 with only minor increase in IL-10 ( Fig. 4c–f ). Thus, while IL-23 supported the Th17 phenotype, IL-27 (and to a lesser extent IL-12) skewed the cytokine production of IL-17 + Th17 cells into a ‘Tr-1’ like phenotype. 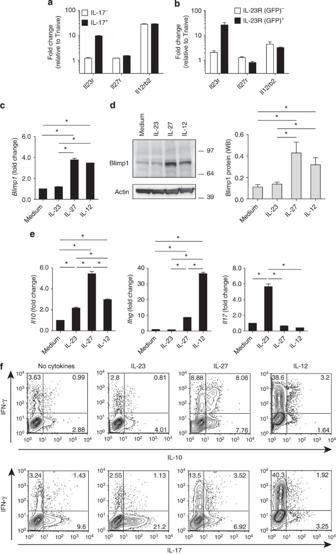Figure 4: IL-27 and IL-12 re-programmebona fideTh17 cells by inducing Blimp1 and IL-10. Sorted IL-17+Th17 cells differentiated with TGF-β plus IL-6 (a) or bona fide Th17 cells (IL-23R (GFP)+CD4+T cells) sorted from the CNS of EAE mice (b) were assessed for the indicated cytokine receptor subunits by quantitative PCR. Mean±s.d.,n=3, representative of two experiments. (c–f) Th17 cells were differentiated from naive wild-type T cells with TGF-β plus IL-6 for 3 days. IL-17-positive cells were separated by an IL-17 secretion assay. After a 6-day-resting phase, cells were re-stimulated without exogenous cytokines or in the presence of IL-23, IL-27 or IL-12 as indicated for 3 additional days. Expression ofBlimp1mRNA as measured by qPCR (c) and Blimp1 protein as measured by western blot (d). Cytokine production in second round T-cell cultures was measured on the mRNA level by qPCR (e) and on the protein level by intracellular cytokine staining (f). Mean±s.d.,n=3, *P<0.05, one-way analysis of variance and Tukey post test, representative of two experiments. Figure 4: IL-27 and IL-12 re-programme bona fide Th17 cells by inducing Blimp1 and IL-10. Sorted IL-17 + Th17 cells differentiated with TGF-β plus IL-6 ( a ) or bona fide Th17 cells (IL-23R (GFP) + CD4 + T cells) sorted from the CNS of EAE mice ( b ) were assessed for the indicated cytokine receptor subunits by quantitative PCR. Mean±s.d., n =3, representative of two experiments. ( c – f ) Th17 cells were differentiated from naive wild-type T cells with TGF-β plus IL-6 for 3 days. IL-17-positive cells were separated by an IL-17 secretion assay. After a 6-day-resting phase, cells were re-stimulated without exogenous cytokines or in the presence of IL-23, IL-27 or IL-12 as indicated for 3 additional days. Expression of Blimp1 mRNA as measured by qPCR ( c ) and Blimp1 protein as measured by western blot ( d ). Cytokine production in second round T-cell cultures was measured on the mRNA level by qPCR ( e ) and on the protein level by intracellular cytokine staining ( f ). Mean±s.d., n =3, * P <0.05, one-way analysis of variance and Tukey post test, representative of two experiments. Full size image In order to test whether the capacity of IL-27 to re-programme committed Th17 cells also applied to in vivo -generated IL-17 producers, we isolated IL-17 + cells by secretion assay from draining lymph nodes of Il23r +/− or Il23r −/− mice that had been immunized with MOG 35-55 in CFA 8 days before. Re-stimulation of these purified in vivo sensitized Th17 cells in the presence of IL-27 resulted in significantly increased expression of Blimp1 and enhanced IL-10 production and a tendency to enhance production of IFN-γ as compared with re-stimulation under neutral conditions ( Fig. 5a,b ). The IL-27-induced increase in IL-10 production was also observed in IL-23R − Th17 cells, which had higher starting levels of IL-10 secretion than IL-23R + Th17 cells. Thus, IL-27 modulated in vivo sensitized Th17 cells to adopt an IL-10-secreting phenotype. 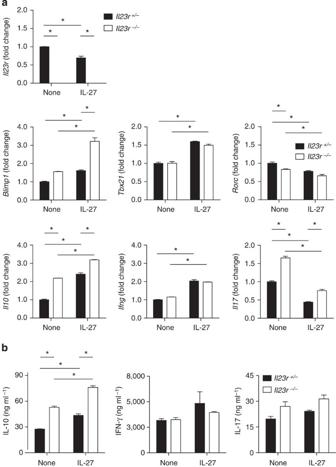Figure 5:In vivocommitted Th17 cells are induced to produce IL-10 by IL-27. Il23r+/−mice andIl23r−/−mice were immunized with MOG35-55in CFA. On day 8, IL-17 producing draining lymph node cells were purified by IL-17 secretion assay. Note that IL-23R-deficient mice were also able to generate IL-17 producing T cells. Wild-type and IL-23R-deficient Th17 cells were rested and re-stimulated without exogenous cytokines or in the presence of IL-27. Second round Th17 cells were assessed for expression of the indicated genes by quantitative RT–PCR (a) and for the secretion of the indicated cytokines by cytometric bead array (b). Mean±s.d.,n=3, *P<0.05, two-way analysis of variance followed by Tukey post test. Figure 5: In vivo committed Th17 cells are induced to produce IL-10 by IL-27. Il23r +/− mice and Il23r −/− mice were immunized with MOG 35-55 in CFA. On day 8, IL-17 producing draining lymph node cells were purified by IL-17 secretion assay. Note that IL-23R-deficient mice were also able to generate IL-17 producing T cells. Wild-type and IL-23R-deficient Th17 cells were rested and re-stimulated without exogenous cytokines or in the presence of IL-27. Second round Th17 cells were assessed for expression of the indicated genes by quantitative RT–PCR ( a ) and for the secretion of the indicated cytokines by cytometric bead array ( b ). Mean±s.d., n =3, * P <0.05, two-way analysis of variance followed by Tukey post test. Full size image Next, we wanted to formally test whether the induction of IL-10 in committed Th17 cells was mediated by Blimp1 and whether IL-27 and IL-12 driven ‘re-programming’ of Th17 cells was dependent on Blimp1. Even under neutral re-stimulation conditions, IL-10 secretion was lower in pre-committed Blimp1-deficient IL-17 + Th17 cells than in wild-type Th17 cells indicating that TcR-driven IL-10 induction in second round cultures depended in part on Blimp1 ( Fig. 6a ). Notably, Blimp1 CKO Th17 failed to reach the same level of IL-10 production as wild-type Th17 cells upon stimulation with either IL-27 or IL-12 while the induction of IFN-γ by IL-27 or IL-12 was not impaired in Blimp1-deficient Th17 cells ( Fig. 6a ). Conversely, when we short circuited cytokine input signalling by ectopically overexpressing Blimp1 in Th17 cells using retroviral transduction, we found strong induction of IL-10 in Th17 cells ( Fig. 6b ). Interestingly, ectopic expression of Blimp1 in Blimp1-deficient Th17 cells increased the fraction of CD49b + Lag-3 + cells, which is a combination of surface markers associated with the Tr-1 phenotype [37] ( Fig. 6c ). Thus, Lag-3 expression appears to be at least in part dependent on Blimp1 expression. Collectively, these data suggested that pre-committed Th17 cells responded to IL-27 (and IL-12) by secreting IL-10 in a Blimp1-dependent manner. 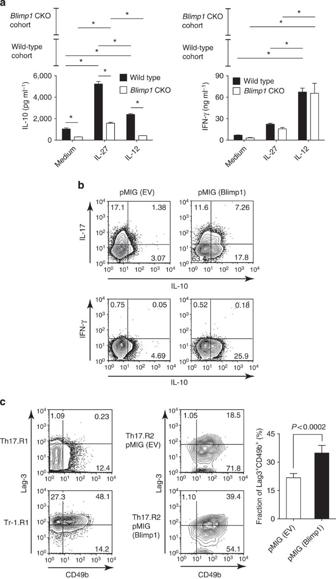Figure 6: Blimp1 is necessary and sufficient to drive IL-10 production in pre-committed Th17 cells. (a,b) Naive CD4+T cells from wild-type orBlimp1CKO mice were differentiated into Th17 cells and sorted for IL-17+T cells by secretion assay. (a) IL-10 and IFN-γ were measured by enzyme-linked immunosorbent assay in the supernatant of second round Th17 cells restimulated as indicated. Mean±s.d.,n=3, *P<0.05, two-way analysis of variance followed by Tukey post test, representative of three experiments. (b) Retroviral overexpression of Blimp1 induces IL-10 in Th17 cells. Th17 cells were differentiatedin vitroand were subsequently transduced with a retroviral vector encoding Blimp1 (pMIG (Blimp1)) or a control vector (pMIG (EV)). Intracellular cytokine staining was performed on day 3 after transduction. Gate on transduced (GFP+) cells. Representative of three experiments. (c) Ectopic overexpression of Blimp1 in Th17 cells increases the fraction of CD49b+Lag-3+double-positive cells.Blimp1CKO T cells were differentiated into Th17 cells and enriched for IL-17 producers by secretion assay. Blimp1-deficient Th17 cells were then transduced with control vector or pMIG (Blimp1) and assessed for CD49b and Lag-3 expression (Th17.R2). Fraction of CD49+Lag-3+cells within the GFP+(transduced) gate. The gates for CD49b and Lag-3 expression were set according to first round Th17 and Tr-1 cells (Th17.R1, Tr-1.R1, left panels). Mean±s.d.,n=3, two-tailedt-test; representative of two experiments. Figure 6: Blimp1 is necessary and sufficient to drive IL-10 production in pre-committed Th17 cells. ( a , b ) Naive CD4 + T cells from wild-type or Blimp1 CKO mice were differentiated into Th17 cells and sorted for IL-17 + T cells by secretion assay. ( a ) IL-10 and IFN-γ were measured by enzyme-linked immunosorbent assay in the supernatant of second round Th17 cells restimulated as indicated. Mean±s.d., n =3, * P <0.05, two-way analysis of variance followed by Tukey post test, representative of three experiments. ( b ) Retroviral overexpression of Blimp1 induces IL-10 in Th17 cells. Th17 cells were differentiated in vitro and were subsequently transduced with a retroviral vector encoding Blimp1 (pMIG (Blimp1)) or a control vector (pMIG (EV)). Intracellular cytokine staining was performed on day 3 after transduction. Gate on transduced (GFP + ) cells. Representative of three experiments. ( c ) Ectopic overexpression of Blimp1 in Th17 cells increases the fraction of CD49b + Lag-3 + double-positive cells. Blimp1 CKO T cells were differentiated into Th17 cells and enriched for IL-17 producers by secretion assay. Blimp1-deficient Th17 cells were then transduced with control vector or pMIG (Blimp1) and assessed for CD49b and Lag-3 expression (Th17.R2). Fraction of CD49 + Lag-3 + cells within the GFP + (transduced) gate. The gates for CD49b and Lag-3 expression were set according to first round Th17 and Tr-1 cells (Th17.R1, Tr-1.R1, left panels). Mean±s.d., n =3, two-tailed t -test; representative of two experiments. Full size image Blimp1 −/− T cells fail to develop into Tr-1 cells in vivo IL-10-deficient mice suffer from enhanced EAE and IL-10 derived from CD4 + Foxp3 − conventional T cells is required for the control of inflammation in the CNS. We hypothesized that Blimp1 could serve as a transcription factor that links the effects of IL-27 (and IL-12) with the induction of IL-10 in conventional T cells under inflammatory conditions in vivo . In order to test the role of Blimp1 as an integrator of IL-12 family cytokine signals, we immunized control mice ( LckCre + × Blimp1 wt/wt ) or mice that conditionally lacked Blimp1 expression in T cells ( Blimp1 CKO) with MOG 35-55 in CFA. Upon ex vivo re-stimulation, CD4 + T cells isolated from the draining lymph nodes of immunized Blimp1 CKO mice showed a severe reduction in IL-10 (and especially IL-10/IFN-γ double) producers as compared with wild-type controls ( Fig. 7a,b ). While the fractions of IFN-γ secreting cells were similar in both groups, Blimp1 CKO mice had increased fractions and absolute numbers of IL-17 producers. Upon standard protocol immunization with MOG 35-55 in CFA, both groups of mice developed EAE, which was somewhat more severe in Blimp1 CKO animals than in controls ( Fig. 7c ). In order to test whether Blimp1 CKO mice were hypersusceptible to EAE, we used a suboptimum EAE induction protocol and compared disease severity and incidence in wild-type and Blimp1 CKO mice ( Fig. 7d ). With this protocol, clinical signs of EAE were not overtly induced in wild-type animals. In contrast, Blimp1 CKO animals developed EAE and showed significantly reduced frequencies of CNS effector CD4 + T cells that produced IL-10 or co-produced IL-10 and IFN-γ ( Fig. 7e ; Supplementary Fig. 3 ). 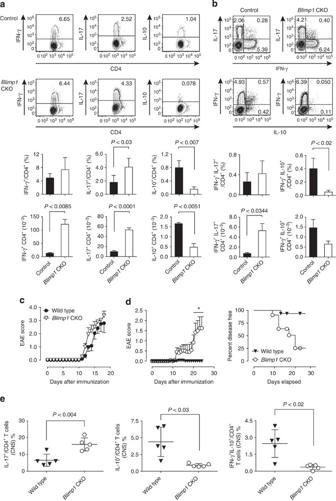Figure 7:Blimp1 is required for the generation of Tr-1-like cellsin vivo. Control mice orBlimp1CKO mice were immunized with MOG35-55in CFA. (a,b) On day 15, draining lymph node cells were stimulatedex vivowith PMA/ionomycin followed by intracellular cytokine staining as indicated. Mean±s.d.,n≥3, two-tailedt-test; representative of two experiments. (c)Blimp1CKO mice develop severe EAE. Lethally irradiated mice were reconstituted with bone marrow of control or T cell conditionalBlimp1CKO mice. After reconstitution, mice were immunized with MOG35-55in CFA plus 200 ng pertussis toxin (PTx) on days 0 and 2 according to the standard EAE induction protocol. Mean EAE scores±s.e.m. are indicated (n=6 per group, representative of two experiments). (d,e) Control mice orBlimp1CKO mice were immunized with MOG peptide in CFA according to a suboptimum regimen (50 ng PTx instead of 200 ng) and followed for signs of disease and disease incidence (d). Mean EAE scores±s.e.m.,n=11, *P<0.05, one-way analysis of variance; representative of two experiments. (e) On day 20 after immunization, the mononuclear infiltrate in the CNS was isolated and infiltrating CD4+T cells were analysed for their cytokine profile by intracellular cytokine staining. Mean±s.d.,n=5, two-tailedt-test; representative of two experiments. Figure 7: Blimp1 is required for the generation of Tr-1-like cells in vivo . Control mice or Blimp1 CKO mice were immunized with MOG 35-55 in CFA. ( a , b ) On day 15, draining lymph node cells were stimulated ex vivo with PMA/ionomycin followed by intracellular cytokine staining as indicated. Mean±s.d., n ≥3, two-tailed t -test; representative of two experiments. ( c ) Blimp1 CKO mice develop severe EAE. Lethally irradiated mice were reconstituted with bone marrow of control or T cell conditional Blimp1 CKO mice. After reconstitution, mice were immunized with MOG 35-55 in CFA plus 200 ng pertussis toxin (PTx) on days 0 and 2 according to the standard EAE induction protocol. Mean EAE scores±s.e.m. are indicated ( n =6 per group, representative of two experiments). ( d , e ) Control mice or Blimp1 CKO mice were immunized with MOG peptide in CFA according to a suboptimum regimen (50 ng PTx instead of 200 ng) and followed for signs of disease and disease incidence ( d ). Mean EAE scores±s.e.m., n =11, * P <0.05, one-way analysis of variance; representative of two experiments. ( e ) On day 20 after immunization, the mononuclear infiltrate in the CNS was isolated and infiltrating CD4 + T cells were analysed for their cytokine profile by intracellular cytokine staining. Mean±s.d., n =5, two-tailed t -test; representative of two experiments. Full size image To test the idea whether lack of Blimp1 in T cells could substitute for IL-23 signalling in T cells regarding their capacity of inducing EAE, we crossed T cell conditional Blimp1-deficient mice onto the Il23r −/− background and immunized them with MOG 35-55 in CFA. Since loss of Blimp1 in T cells does not reduce (but rather increases) IFN-γ production (see for example Fig. 3b ), we treated control Il23r −/− mice and Il23r −/− × Blimp1 CKO mice with a neutralizing monoclonal antibody to IFN-γ. Notably, while Il23r −/− animals remained resistant to EAE, Il23r −/− × Blimp1 CKO mice became sick ( Supplementary Fig. 4 ) suggesting that IL-23 signalling is dispensable for conferring encephalitogenic properties to Blimp1-deficient T cells. Taken together, these data indicated that Blimp1 was required for inducing IL-10 production in conventional CD4 + T cells under inflammatory conditions, thus relaying signals from IL-27/IL-12 vs IL-23 for T cell intrinsic regulation of inflammation. In the present study, we demonstrate that in the absence of IL-10 and IFN-γ double producing T cells, IL-23 is dispensable for autoimmune pathology. We define the transcriptional regulator Blimp1 as a major transcription factor that mediates signals from the IL-12 family cytokines IL-27 and IL-12 to promote the generation of IL-10 and IFN-γ producing conventional T cells (Tr-1-like cells) in the context of autoimmune CNS inflammation. The balance of IL-23 on one hand vs IL-12 and IL-27 on the other hand can be sensed by Th17 cells. Th17 cells then integrate these signals into graded upregulation of Blimp1. The higher the expression of Blimp1, the more Th17 cells lose their pathogenic identity and adopt an IL-10 and IFN-γ-producing Tr-1-like phenotype that contributes to resolving rather than promoting inflammation. Both CD4 + and CD8 + T cells are increasingly being recognized as important sources of IL-10 to limit immunopathology in an effector T-cell intrinsic manner in infectious and autoimmune inflammatory conditions [13] , [23] , [38] , [39] . Conventional CD4 + T cells that produce IL-10 and IFN-γ have been called Tr-1 cells [10] . IL-27 (together with TGF-β) was identified to induce the transcription factor c-Maf, which cooperates together with Ahr to drive the production of IL-10 in these cells [36] . c-Maf was found to directly bind to the Il-10 promoter and c-Maf-deficient CD4 + T cells failed to produce IL-10 in response to IL-27 (ref. 16 ). Yet, c-Maf is not unique to the Tr-1 signature since it is also expressed in Th2 (ref. 40 ) and Th17 cells [34] . Th17 cells and Tr-1 cells differ in their ability to produce IL-10. Thus, we hypothesized that besides c-Maf and Ahr , additional regulators must be operational to drive IL-10 in Tr-1 cells. Here, we screened for transcription factors differentially expressed between Tr-1 and Th17 cells and found that Blimp1 was expressed in Tr-1 but not in Th17 cells. We demonstrate that the production of IL-10 from antigen-specific conventional CD4 + T cells under inflammatory conditions in vivo is dependent on Blimp1 induction by IL-12 family cytokines, namely IL-12 and IL-27. In contrast, IL-10 production in the presence of TGF-β signals does not depend on Blimp1 but requires c-Maf and Ahr, indicating the existence of Blimp1-dependent and -independent ways of IL-10 induction—perhaps reflecting the possibility to initiate IL-10 production in the context of distinct ambient cytokine milieus. Blimp1-mediated induction of IL-10 is highly relevant in pre-committed CD4 + effector T cells at sites of active inflammation. The majority of effector T helper cells recruited to the CNS during autoimmune inflammation are current or former Th17 cells [6] and express both subunits of the IL-12R and IL-27R [41] . Here, we show that IL-27 (and IL-12) but not IL-23 induce Blimp1 expression in purified bona fide IL-17 secreting Th17 cells irrespective of whether they were differentiated in vitro or in vivo . Exposure to IL-27 or IL-12 results in the re-programming of Th17 cells into IL-10 and IFN-γ producing Tr-1-like cells. A previous report suggested that IL-27 had limited effect on the suppression of IL-17 production and induction of IL-10 in pre-committed Th17 cells [42] . However, bulk cultures and not sorted IL-17 producers were used for in vitro second round stimulations in this study. IL-27 leads to phosphorylation of Stat1 and Stat3 in Th17 cells [42] . Interestingly, IL-21 can induce IL-10 expression in CD4 + and CD8 + T cells in a Stat3-dependent manner [43] . Coupled with the observation that IL-21 can also promote expression of Blimp1 in activated B cells, CD4 + T cells and CD8 + T cells [44] , these data suggest that Stat3 signals can induce IL-10 production in a Blimp1-dependent manner. In Th17 cells, IL-12 signalling results in phosphorylation of Stat4 ( Supplementary Fig. 5 ), which directly binds to regulatory elements in the Blimp1 gene ( Supplementary Fig. 5 ). In turn, ectopic expression of Blimp1 in Th17 cells results in the secretion of IL-10. Thus, we propose that IL-27 and IL-12 initiate a cascade of re-programming events that converge in changing pathogenic Th17 cells into Tr-1-like cells. Similarly, IL-12-induced expression of Blimp1 is required for Th1 cells to acquire an IL-10-producing phenotype. Thus, ‘Tr-1’ cells may be conceptualized as Blimp1-dependent developmental end-stage of distinct effector T helper cells rather than a lineage of their own, and Blimp1 expression emerges as a nodal point in the control of this fate decision event. The in vivo importance of IL-27 (and IL-12) re-programmed effector T helper cells was demonstrated by our observation that genetic disruption of the IL-27 (and IL-12) target genes Il-10 and Ifng promoted fulminant inflammation in a model of T cell-mediated autoimmunity of the CNS even in the absence of IL-23R signalling. IL-27R and IL-12Rβ2-deficient mice have previously been reported to develop more severe EAE, which has been attributed to decreased production of IL-10 and IFN-γ by effector T helper cells, respectively [45] , [46] . IL-10 has long been known as anti-inflammatory cytokine in EAE [47] , [48] . Although IFN-γ has pro-inflammatory properties [49] , it also contributes to the resolution of inflammatory infiltrates in later disease stages via its anti-proliferative and proapoptotic effects [46] , [50] . Here, we propose that the balance between upstream IL-27 (and IL-12) vs IL-23 cytokine signalling into the same pre-committed T cell determines its production of IL-10 and IFN-γ vs IL-17 and GM-CSF via the extent of Blimp1 induction. Accordingly, increased frequencies of Th17 cells have been reported in mice with T cell conditional deficiency of Blimp1 in models of colitis and type 1 diabetes [51] , [52] . This concept places T-cell subsets, such as Th17 cells, which can respond to both sets of IL-12 family cytokines in a key position for determining the outcome of inflammatory processes. In fact, the IL-23/IL-17 axis is unmasked to be dispensable for T helper cell intrinsic pathogenicity when the counterregulatory IL-27, IL-12/Blimp1/IL-10 pathway is abrogated. Thus, therapeutic interventions of ongoing T cell-mediated immunopathology should—by design—attenuate the IL-23/IL-17 axis and strengthen the IL-27, IL-12/Blimp1 axis. Our data may explain why treatment of multiple sclerosis with a monoclonal antibody to p40, which blocks IL-23 and IL-12 at the same time, failed to be successful and had an even net effect on the inflammatory disease activity [53] . In summary, this study provides a potential transcriptional framework for T helper cell intrinsic plasticity in an inflammatory context. There is an urgent need to further advance the molecular understanding of late re-programming events in antigen-specific T cells, because therapeutic interventions will have to be effective in ongoing and not only nascent organ-specific autoimmunity. Mice All mouse strains were generated on a C57BL/6 genetic background or backcrossed onto the C57BL/6 genetic background for at least 10 generations. Mice were bred in specific pathogen-free facilities at the Klinikum rechts der Isar of the Technical University Munich or at the Walter and Eliza Hall Institute of Medical Research, Parkville. All experimental protocols were approved by the standing committee for experimentation with laboratory animals of the Bavarian state authorities (AZ 55.2-1-54-2531-88-08 and AZ 55.2-1-54-2532-164-11) or the animal ethics committee of the Walter and Eliza Hall Institute and performed in accordance with the corresponding guidelines. IL-23R reporter mice ( Il23r gfp/+ ) harbour an Il23r allele that is disrupted by an inserted internal ribosome entry site-GFP (green fluorescent protein) cassette [28] . Homozygous mice of this strain are IL-23R deficient and were designated Il23r −/− mice. Foxp3gfp knock-in mice [8] , Blimp1 reporter mice ( Blimp1 gfp/+ ) [54] and T cell conditional Blimp1 KO mice ( Lck Cre or CD4 Cre × Blimp1 flox/flox ) [55] , [56] were described before. Il-10 −/− mice [57] and Ifng −/− mice [49] were obtained from Jackson laboratories (Bar Harbor). Sex-matched mice were used for experiments at 6–8 weeks of age. Induction of EAE EAE was induced by subcutaneous immunization in the base of tail with 200 μg of MOG 35-55 (MEVGWYRSPFSRVVHLYRNGK; Auspep, Tullamarine, Australia) in complete Freund’s adjuvant containing 500 μg Mycobacterium tuberculosis H37Ra (Difco) per mouse plus intravenous injection of 200 ng pertussis toxin (Sigma-Aldrich) on days 0 and 2 after immunization (standard protocol). For suboptimum EAE induction, mice received reduced amounts of pertussis toxin (50 ng) on days 0 and 2 after immunization. For generation of bone marrow chimeric mice, Rag1 −/− mice were irradiated with 2 × 3.3 Gy. On the next day, recipient mice were injected with equal amounts of T-cell-depleted (CD90.2 microbeads, Miltenyi) bone marrow cells (6 × 10 6 each). After a reconstitution period of at least 4 weeks, mice were immunized with MOG 35-55 in CFA. Disease progress and severity were assessed as described [39] . The peak of disease was typically between 15 and 20 days post immunization with the standard protocol. Preparation of mononuclear cells from the CNS Mice were perfused through the left cardiac ventricle with phosphate-buffered saline. The forebrain and cerebellum were dissected and spinal cords flushed out with phosphate-buffered saline by hydrostatic pressure. CNS tissue was cut into pieces and digested with 2.5 mg ml −1 collagenase D (Roche Diagnostics) and 1 mg ml −1 DNaseI (Roche Diagnostics) at 37 °C for 45 min. Mononuclear cells were isolated by passing the CNS tissue through a 70 μm cell strainer (BD Biosciences), followed by a percoll gradient (70%/37%) centrifugation. The cells were removed from the interphase, washed and resuspended in culture medium for further analysis. T-cell culture Cells were cultured in DMEM (PAA) supplemented with 10% fetal calf serum, 5 × 10 −5 M β-mercaptoethanol, 1 mM sodium pyruvate, non-essential amino acids, L -glutamine, 100 U ml −1 penicillin and 100 μg ml −1 streptomycin. For in vitro T-cell differentiation, magnetic bead-purified CD4 + CD62L + (Miltenyi) or flow cytometrically purified CD4 + CD44 − CD25 − T cells were stimulated for 3 days with 4 μg ml −1 plate-bound antibody to CD3 (BioXcell, 145-2C11) and 2 μg ml −1 soluble antibody to CD28 (BioXcell, PV-1). Recombinant cytokines were obtained from R&D systems. If not otherwise indicated, Th1 cells were differentiated in the presence of 10 ng ml −1 IL-12 and 10 μg ml −1 anti-IL-4 (11B11, BioXcell), Th17 cells were differentiated in the presence of 0.5 ng ml −1 TGF-β1 and 50 ng ml −1 IL-6 and Tr-1 cells were differentiated with 0.5 ng ml −1 TGF-β1 and 100 ng ml −1 IL-27. Bona fide IL-17 secreting cells were isolated using a magnetic bead based IL-17 secretion assay (Miltenyi) according to the manufacturer’s instructions. For re-stimulation cultures, T cells were rested for 5–6 days in the presence of IL-2 (2 ng ml −1 ) before re-stimulation in the presence of IL-12, IL-23 or IL-27 (10 ng ml −1 ). Intracellular cytokine staining For ICCS, cells were isolated and stimulated in culture medium containing 50 ng ml −1 PMA, 1 μg ml −1 ionomycin (both Sigma-Aldrich) and 1 μl ml −1 GolgiStop (monensin, BD Biosciences) at 37 °C and 5% CO 2 for 3 h. After live/dead staining with Aqua dead cell stain (Invitrogen), cells were stained for surface markers (CD3 (145-2C11; BD Biosciences), CD4 (RM4-5; BD Biosciences), CD49b (HMa2, BioLegend), and Lag-3 (C9B7W, eBioscience)). Subsequently, cells were fixed and permeabilized (Cytofix/Cytoperm and Perm/Wash buffer, BD Biosciences) followed by staining with monoclonal antibodies to mouse IL-17A (TC11-18H10.1; BioLegend), IL-10 (JES5-16E3; BD Bioscience), IFN-γ (XMG1.2; eBioscience) and GM-CSF (MP1-22E9; BD Bioscience). All antibodies were used 1:100, except for IFN-γ (1:200). For Foxp3 detection, the Foxp3 staining kit from eBioscience was used according to the manufacturer’s recommendation. Cells were measured on a CyAn ADP Machine (Beckman Coulter) and flow cytometric data analysis was performed with FlowJo software (TreeStar, Ashland, OR). Quantitative PCR analysis and enzyme-linked immunosorbent assay RNA was extracted using RNeasy columns (Qiagen). In some experiments RNA was extracted from fixed cells using the RNeasy FFPE procedure (Qiagen). Complementary DNA (cDNA) was transcribed as recommended (Applied Biosystems) and used as template for qPCR. Primer plus probe mixtures were obtained from Applied Biosystems. The TaqMan analysis was performed using a OneStepPlus system (Applied Biosystems). Gene expression was normalized to the expression of β-Actin (Applied Biosystems). Secretion of IL-10, IL-17 and IFN-γ was detected by standard sandwich enzyme-linked immunosorbent assay (R&D Systems, DuoSet) or cytometric bead array (eBioscience). Standard curves and sample concentrations were calculated based on the mean of triplicates for each dilution or sample. Western blot After in vitro differentiation, T cells were lysed and denatured using RIPA buffer (Sigma-Aldrich) supplemented with protease inhibitor (Sigma). The protein lysates were separated by SDS–PAGE in 4–12% NuPAGE Bis-Tris Mini gels and transferred to nitrocellulose membranes (Invitrogen). After blocking with 5% low-fat dry milk in TBS-T, membranes were incubated with primary antibodies to Blimp1 (5E7, Santa Cruz; 1:50), or β-Actin (Abcam; 1:2,500) in blocking solution overnight at 4 °C. Primary antibody binding was detected with HRP-conjugated secondary antibodies (Dianova; 1:10,000). The signal was visualized by enhanced chemiluminescence (Novex ECL, Invitrogen) and analysed by densitometric scanning of exposed X-ray films (GE Healthcare) or by Fusion SL blot documentation equipment (Peqlab). Retroviral transduction of T cells A retroviral construct was generated by cloning of full-length mouse Blimp1 cDNA (Open Biosystems/Thermo Scientific, clone 40048956) via EcoRI and XhoI into the retroviral internal ribosome entry site-containing vector pMIG II [58] , allowing the bicistronic co-expression of Blimp1 and GFP. Cells of the retrovirus producer line Phoenix-Eco (kind gift of Hans-Martin Jäck, Erlangen) were transiently transfected with plasmids (Blimp1 pMIG II or control pMIG II empty vector) by calcium phosphate precipitation in the presence of 25 μM chloroquine (Sigma-Aldrich). Retroviral supernatants were collected 2 days after transfection. T cells were transduced 24 h after polyclonal in vitro activation of naïve sorted CD4 + T cells with TGF-β and IL-6 (Th17). Retroviral supernatant and 4 μg ml −1 polybrene (Merck Millipore) were added to the pre-committed T cells and a spin transduction was performed (2,000 r.p.m., room temperature, 1 h). Cells were further cultured for 3 days in polarizing conditions before analysis by intracellular cytokine staining. Microarray platform Total RNA was isolated from five independent samples of in vitro- differentiated Th0, Th17 and Tr-1 cells (d3) using RNeasy Mini Kit (Qiagen). RNA quality was tested on a Bioanalyzer. Using the Ambion WT expression kit, two cycles of cDNA synthesis were performed. Single-stranded cDNA was fragmented and labelled with biotin allonamide triphosphate using the GeneChip WT terminal labelling kit. Five micrograms of fragmented and labelled cDNA were hybridized to the GeneChip Mouse Gene 1.0 ST Array at the Institute for Microbiology of the Technical University Munich (Munich, Germany). Data analysis was performed using GenePattern open source software ( www.genepattern.broadinstitute.org ). Statistical analysis Statistical evaluations of cell frequency measurements, cell numbers, messenger RNA and protein levels were performed with the unpaired Student’s t -test when two populations were compared. Two-tailed P -values <0.05 were considered significant. Multiple comparisons were performed with one-way analysis of variance followed by post hoc test (Tukey). EAE scores between groups were analysed as disease burden per individual day with one-way analysis of variance and post hoc test as indicated. Accession codes: Microarray data have been deposited in the Gene Expression Omnibus database under accession code GSE56021 . How to cite this article: Heinemann, C. et al. IL-27 and IL-12 oppose pro-inflammatory IL-23 in CD4 + T cells by inducing Blimp1. Nat. Commun. 5:3770 doi: 10.1038/ncomms4770 (2014).